Guidance of subcellular tubulogenesis by actin under the control of a synaptotagmin-like protein and Moesin Apical membranes in many polarized epithelial cells show specialized morphological adaptations that fulfil distinct physiological functions. The air-transporting tubules of Drosophila tracheal terminal cells represent an extreme case of membrane specialization. Here we show that Bitesize (Btsz), a synaptotagmin-like protein family member, is needed for luminal membrane morphogenesis. Unlike in multicellular tubes and other epithelia, where it influences apical integrity by affecting adherens junctions, Btsz here acts at a distance from junctions. Localized at the luminal membrane through its tandem C2 domain, it recruits activated Moesin. Both proteins are needed for the integrity of the actin cytoskeleton at the luminal membrane, but not for other pools of F-actin in the cell, nor do actin-dependent processes at the outer membrane, such as filopodial activity or membrane growth depend on Btsz. Btsz and Moesin guide luminal membrane morphogenesis through organizing actin and allowing the incorporation of membrane containing the apical determinant Crumbs. The tubes that transport liquids and gases through animal bodies are composed of multicellular epithelia or they can be fine, subcellular tubes. The establishment and maintenance of an apical plasma membrane domain is essential for the creation of the tube lumen [1] , [2] , [3] , [4] , [5] , [6] , [7] . In multicellular tubes, the definition of the apical domain is closely associated with the integrity of apical adherens junctions. In subcellular tubes, which may be shaped either by cell hollowing or by elongation of a membrane invagination, tube morphogenesis can occur in the absence of or at a great distance from cell junctions. This is the case in de novo angiogenesis in vertebrates, in the excretory cell in C. elegans and in the terminal cells of the oxygen-transporting tracheal system in insects [8] , [9] , [10] , [11] , [12] , [13] . The tube lumen in the terminal cell of the Drosophila tracheal system begins to grow late in embryogenesis from the site at which the cell is connected to a multicellular tracheal branch [14] , [15] , but most of its elongation occurs during the extensive body growth of the third instar larva. Molecules involved in the growth of tracheal branches and the formation of the subcellular lumen include proteins typically associated with apical plasma membranes, several of which localize at the luminal membrane [2] , [16] , [17] , [18] , [19] , as well as the microtubule [1] , [20] , [21] and the actin cytoskeleton. Actin filaments are present at the growing tip of terminal cells, at the outer, basal plasma membrane and at the luminal membrane, and actin-regulating molecules such as SRF, Ena, IKK ͛ and Talin contribute to tracheal cell morphogenesis [1] , [21] , [22] , [23] , [24] . The connection between the basal actin network with the outer plasma membrane in larval terminal cells is made through Talin, which links the network to the extracellular matrix via the integrin complex, and this link is required for proper tube morphology [24] . Filopodial function requires Ena [21] , but how the growing luminal membrane interacts with the actin cytoskeleton and which actin regulators might be involved in larval tube morphogenesis are unknown. Here we show that the protein Bitesize (Btsz) regulates the luminal actin cortex of terminal cells. This is mediated by the interaction between Btsz and Moesin through the Moesin binding domain (MBD) of Btsz and is independent of its function in stabilizing the adherens junctions. Furthermore, we find that Btsz-mediated organization of the luminal cortex guides the delivery of a specific subset of apically targeted cargo that includes the transmembrane protein Crumbs. Role of Btsz in terminal cell development We had found that the gene btsz , identified in a screen for messenger RNAs (mRNAs) localized in terminal branches, is required for terminal cell morphogenesis [25] . Btsz is the only Drosophila member of the family of synaptotagmin-like proteins (SLPs) [26] , [27] , which play important roles in multicellular epithelial tubes [28] , [29] . Two independently-derived mutant alleles of btsz have been reported [26] , [27] . btsz J5-2 homozygous mutants die early during embryogenesis, while btsz K13-4 mutants survive to late larval or pupal stages, with a range of defects in terminal tracheal cells ( Fig. 1b,d ). Terminal cells had reduced number of branches and defects in tube morphogenesis, such as multiple, thin parallel luminal structures within the cell body or irregularly shaped lumens ( Fig. 1b,d ). Transheterozygotes and larvae expressing an RNA interference (RNAi) construct showed a similar phenotype ( Supplementary Fig. S1C,D ). Therefore, the observed defects were due to mutations in btsz , and btsz acts in a cell-autonomous manner specifically in tracheal cells. 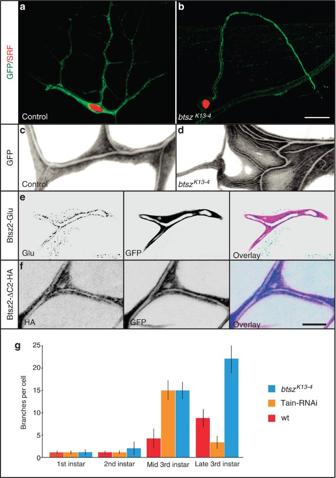Figure 1: Phenotype of terminal cells inbtszK13-4mutant larvae and subcellular localization of Btsz. (a–d) Overview and details of control (a,c) andbtszK13-4mutant (b,d) terminal cells in third instar larvae. (a,b) The terminal cell nuclei are visualized by immunostaining with antibodies against SRF (red) and the cells are labelled with cytoplasmic GFP (green).btszK13-4mutant terminal cells have fewer or no branches compared with control. (c,d) High magnification details of terminal cells shown in inverted colour or grey scale for better clarity. (c) In the control cell, a single lumen is present in each branch. (d) Example of a mutant cell containing many parallel, thin lumens emanating from a larger lumen. (e,f) Subcellular localization of Btsz. Single focal plane details of terminal branches expressing cytoplasmic GFP and tagged Btsz proteins, visualized by staining with antibodies against the tags. The connections of the part of the cell shown in the image to the rest of the cell is in a different focal plane. Btsz2-Glu (e) has the C2 domains and localizes to the apical membrane. Btsz2-ΔC2-HA (f) lacks the exons encoding the C2 domains and the encoded protein is distributed throughout the cytoplasm. The staining seen outside the terminal branch ineis background staining by the Anti-Glu antiserum, which is also seen in the absence of the Btsz2-Glu transgene. Images (a–d) are projections of confocal image stacks and (e,f) are single focal planes. Scale bars: (a,b) 50 μm and (c–f) 10 μm. (g) Terminal cell branching during larval development. Larvae expressing UAS-GFPbtl-Gal4 were analysed at the indicated ages. The number of branches in dorsal terminal cells in tracheal segments tr2 to tr9 were counted (n>10 for each genotype and time point, error bars represent s.d.). GFP, green fluorescent protein. Figure 1: Phenotype of terminal cells in btsz K13-4 mutant larvae and subcellular localization of Btsz. ( a – d ) Overview and details of control ( a , c ) and btsz K13-4 mutant ( b , d ) terminal cells in third instar larvae. ( a , b ) The terminal cell nuclei are visualized by immunostaining with antibodies against SRF (red) and the cells are labelled with cytoplasmic GFP (green). btsz K13-4 mutant terminal cells have fewer or no branches compared with control. ( c , d ) High magnification details of terminal cells shown in inverted colour or grey scale for better clarity. ( c ) In the control cell, a single lumen is present in each branch. ( d ) Example of a mutant cell containing many parallel, thin lumens emanating from a larger lumen. ( e , f ) Subcellular localization of Btsz. Single focal plane details of terminal branches expressing cytoplasmic GFP and tagged Btsz proteins, visualized by staining with antibodies against the tags. The connections of the part of the cell shown in the image to the rest of the cell is in a different focal plane. Btsz2-Glu ( e ) has the C2 domains and localizes to the apical membrane. Btsz2-ΔC2-HA ( f ) lacks the exons encoding the C2 domains and the encoded protein is distributed throughout the cytoplasm. The staining seen outside the terminal branch in e is background staining by the Anti-Glu antiserum, which is also seen in the absence of the Btsz2-Glu transgene. Images ( a – d ) are projections of confocal image stacks and ( e , f ) are single focal planes. Scale bars: ( a , b ) 50 μm and ( c – f ) 10 μm. ( g ) Terminal cell branching during larval development. Larvae expressing UAS-GFP btl- Gal4 were analysed at the indicated ages. The number of branches in dorsal terminal cells in tracheal segments tr2 to tr9 were counted ( n >10 for each genotype and time point, error bars represent s.d.). GFP, green fluorescent protein. Full size image When expressed in tracheal cells, a tagged Btsz construct (Btsz2-Glu), which localizes apically in the ovarian follicle epithelium and at the adherens junctions in the blastoderm epithelium [26] , [27] , is found throughout the length of the terminal branches, localizing at the luminal membrane ( Fig. 1e ). This distribution depends on the tandem C2 domain, since a construct lacking this part (Btsz2-ΔC2-HA) is distributed more evenly throughout the cytoplasm ( Fig. 1f ). To understand how Btsz contributes to the formation of tubes and branches, we first assessed when the btsz defects manifest and how they progress during larval development. Terminal cells begin to branch in the second instar, adding most branches in the third larval instar, with averages of 15 and 24 branches per cell at the two time points of counting ( Fig. 1g ; Supplementary Fig. S2A–F ). btsz K13-4 terminal cells go from 4.25 to 8.33 branches at the same time points. Loss of Talin, previously shown to be needed for branch and tube morphogenesis, has a different effect. While the cells begin to grow the same number of branches as control cells in the mid-third instar, they end up with an average of only 3.4 branches per cell at late third instar, confirming earlier reports that branches are made, but then disappear [24] . Thus, while Talin-depleted cells can form branches, but these are unstable, Btsz-depleted cells fail to develop branches in the first place. Btsz requirement for luminal versus outer membrane morphogenesis The fact that we observe both a loss of branches and luminal defects raises the question whether the primary function of Btsz is to allow luminal membrane formation—as suggested by its subcellular localization—with the lack of branches being a secondary effect. Alternatively, Btsz could be needed primarily for branch formation, or it may have independent roles in both processes. It is possible that if newly formed branches do not succeed in elaborating a lumen, they will not be stabilized or continue to grow. Short new branches or short extensions of existing branches without lumen can be found in larval terminal cells ( Supplementary Fig. S2G ), but never long, tubeless branches. Consistent with the notion that branch growth persists over longer distances only when a lumen is formed following initial branch outgrowth, no mutants have been discovered in which third instar branches completely lack a lumen (although final lumen maturation is not a condition for branches to persist [1] , [2] , [30] ). To distinguish between a requirement of Btsz for lumen or branch formation, live observations are necessary, but they are not possible for extended periods in the larva. We therefore analysed terminal cell growth in embryos. We imaged two fluorescent reporters, the PtdIns(4,5)P2 sensor PLCδ-PH-GFP as a marker for the apical membrane, and the actin-binding domain of Utrophin fused to GFP (Ut-ABD-GFP) ( Fig. 2a,c and Supplementary Movies 1,2 ). PLCδ-PH-GFP is present at low levels throughout the whole cell and is strongly enriched at the luminal membrane. Actin is seen in the filopodial protrusions extending from the migrating tip and other parts of the cell, and later, in association with the lumen of the cell. With both reporters, the luminal membrane becomes visible when the cell has a length of ~15 μm; it then grows at the same rate as the cell. In terminal cells with reduced Btsz levels, the filopodial activity of the leading tip appeared normal, and branch extension occurred ( Fig. 2b,d ; Supplementary Movies 3,4 ). However, the lumen did not follow the tip of the cell at the normal distance; it lagged behind or formed ectopic branches. Some cells had no lumen at all, even though they had produced extensive filopodia, the growth of the outer, basal plasma membrane was not impaired and the branch grew to its normal length ( Supplementary Movie 5 ). The further development of such tubeless cells cannot be imaged because the embryos begin to move. We observed no defects in terminal cells in which Talin had been reduced by RNAi ( Supplementary Movie 6 ). A quantitative comparison of the ratio of lumen-to-cell length in staged and fixed embryos showed that the lumen was on average 64% of the length of the cell in Btsz-depleted cells compared with an average of 88% in the control cells ( Fig. 2e ). In summary, Btsz is specifically required for the morphogenesis of the inner tube membrane and not for the growth of the branch per se . We conclude that the lack of branches in the larva is most likely a secondary consequence of a failure in lumen formation. 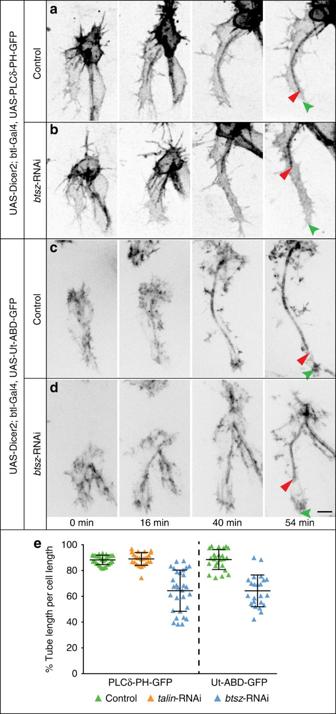Figure 2: Defects in terminal cell lumen formation in Btsz-depleted embryos. Snap shots from time-lapse movies of the development of dorsal terminal cells in the embryo. (a,c) Terminal cells from control embryos expressing Dicer2 together with PLCδ-PH-GFP (a) or Ut-ABD-GFP (c). (b,d) Embryos expressingbtsz-RNAi in addition to Dicer2 and the reporter constructs. The red arrowhead marks the tip of the lumen, the green arrowhead marks the leading edge of the cell. (e) Ratio of lumen-to-cell length in control, Btsz- and Talin-depleted embryos. At stage 16–17, the average tube length in control embryos was 88% (±3.5) and 88.5% (±7.7) of the length of the cell in PLCδ-PH-GFP- and Ut-ABD-GFP-expressing embryos, respectively. In Btsz-depleted cells, the average tube length was reduced to 64.4% (±16) and 64.3% (±12.4), respectively (P<0.001 in both cases by two-tailedt-test). Knockdown of Talin did not lead to a reduction in the tube-to-cell ratio (89.1%±5), (n>20 for each cross ine, error bars represent s.d.). Scale bar: (a–d) 5 μm. GFP, green fluorescent protein. Figure 2: Defects in terminal cell lumen formation in Btsz-depleted embryos. Snap shots from time-lapse movies of the development of dorsal terminal cells in the embryo. ( a , c ) Terminal cells from control embryos expressing Dicer2 together with PLCδ-PH-GFP ( a ) or Ut-ABD-GFP ( c ). ( b , d ) Embryos expressing btsz -RNAi in addition to Dicer2 and the reporter constructs. The red arrowhead marks the tip of the lumen, the green arrowhead marks the leading edge of the cell. ( e ) Ratio of lumen-to-cell length in control, Btsz- and Talin-depleted embryos. At stage 16–17, the average tube length in control embryos was 88% (±3.5) and 88.5% (±7.7) of the length of the cell in PLCδ-PH-GFP- and Ut-ABD-GFP-expressing embryos, respectively. In Btsz-depleted cells, the average tube length was reduced to 64.4% (±16) and 64.3% (±12.4), respectively ( P <0.001 in both cases by two-tailed t -test). Knockdown of Talin did not lead to a reduction in the tube-to-cell ratio (89.1%±5), ( n >20 for each cross in e , error bars represent s.d.). Scale bar: ( a – d ) 5 μm. GFP, green fluorescent protein. Full size image Interaction of Btsz with Moesin at the luminal actin cortex Previously reported roles for Btsz have involved its influence on the stability of adherens junctions [27] , [29] . Terminal cells have adherens junctions only at their base, where they are connected to the primary unicellular branch. This junction is difficult to image, and the junctional E-cadherin is not always detectable even in control cells ( Fig. 3a,b ). However, a proper junction was seen in many btsz K13-4 mutant terminal cells that had serious branching defects ( Fig. 3c ), showing that failure to form a proper tube does not correlate with defects in the junction. The only other defects in adherens junctions in the tracheal system in btsz K13-4 larvae were seen in the fusion cells of the dorsal trunk, where the junction that forms de novo between the two fusion cells is often fragmented or not detectable ( Fig. 3e,f ; Supplementary Movies 7,8 ). 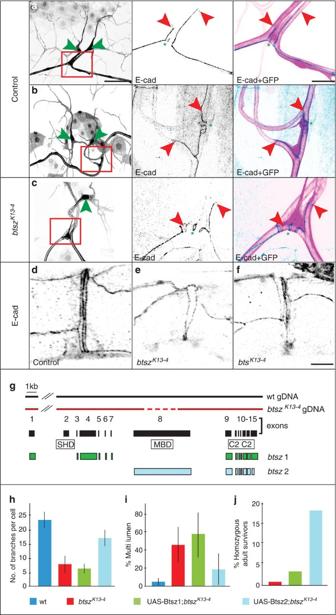Figure 3: Adherens junctions and role of the MBD of Btsz in terminal cells. (a,b) E-cadherin (E-cad) in control and inbtszK13-4mutant (c) dorsal terminal cells in third instar larvae. Junctions are seen, both in control and mutant larvae, at the site where the terminal cell is joined to the dorsal branch (red arrowheads) and between the two dorsal fusion cells (asterisk) as well as along the length of the unicellular junction in the dorsal branch cell. Compare (a) and (b) for variability in expression of E-cad in control junctions. Nuclei of the terminal cells in the low-magnification panels (a–c) are marked with green arrowheads. E-cad-stained control (d) andbtszK13-4mutant (e,f) fusion cells that connect the segmental units of the dorsal trunk in the third instar larva. 4,6-diamidino-2-phenylindole staining to visualize nuclei confirms that two cells are present (seeSupplementary Movie 8). (g) Schematic of thebtsztranscription unit and two of the alternative transcripts (adapted from Serranoet al.26). The wild type and thebtszK13-4genomic regions are represented as lines with the dashed region indicating the deletion in thebtszK13-4allele. Boxes below represent the 15 exons ofbtsz(black) and the organization of exons inbtsztranscripts 1 (green) and 2 (blue). (h–j) Ability ofbtsztransgenes to suppress defects inbtszK13-4mutants. The indicated transgenic constructs were expressed in the tracheal system ofbtszmutant animals and various aspects of thebtszmutant phenotype were scored. The colours of the bars correspond to those in the diagram above. Genotypes of crosses and number of larvae scored: red:btl-GAL4, UAS-GFP;btszK13-4/TM6B, Tb (n=17). Green:btl-GAL4, UAS-GFP;btszK13-4/TM6B, Tb X UAS-Btsz1;btszK13-4/TM6B, Tb (n=18). Blue:btl-GAL4, UAS-GFP;btszK13-4/TM6B, Tb X UAS-Btsz2;btszK13-4/TM6B, Tb (n=15). Error bars inhandirepresent s.d.. Btsz2, but not Btsz1, suppresses the defects in branching (h) and the multi-lumen phenotype (i) ofbtszK13-4homozygous mutants (P=5.5 × 10−7and 5.6 × 10−5respectively, by two-tailedt-test). (j) Ability of the same transgenes to suppress lethality of homozygousbtszK13-4adults. If lethality ofbtszK13-4were completely suppressed, the expected proportion of homozygous mutant flies among the offspring of the cross would be 33% (the remaining 66% are heterozygous for the balancer chromosome; homozygous balancer animals die in early larval instars). Thus, about half of the mutants were rescued to viability by the transgene. Images (a–f) are projections of confocal image stacks. Scale bars: (a–cleft) 75 μm and (a–cmiddle and right,d–f) 20 μm. C2, region encoding the tandem C2 domains; GFP, green fluorescent protein; MBD, region encoding the Moesin binding domain; SHD, region encoding a Synaptotagmin-like-protein homology domain. Figure 3: Adherens junctions and role of the MBD of Btsz in terminal cells. ( a , b ) E-cadherin (E-cad) in control and in btsz K13-4 mutant ( c ) dorsal terminal cells in third instar larvae. Junctions are seen, both in control and mutant larvae, at the site where the terminal cell is joined to the dorsal branch (red arrowheads) and between the two dorsal fusion cells (asterisk) as well as along the length of the unicellular junction in the dorsal branch cell. Compare ( a ) and ( b ) for variability in expression of E-cad in control junctions. Nuclei of the terminal cells in the low-magnification panels ( a – c ) are marked with green arrowheads. E-cad-stained control ( d ) and btsz K13-4 mutant ( e , f ) fusion cells that connect the segmental units of the dorsal trunk in the third instar larva. 4,6-diamidino-2-phenylindole staining to visualize nuclei confirms that two cells are present (see Supplementary Movie 8 ). ( g ) Schematic of the btsz transcription unit and two of the alternative transcripts (adapted from Serrano et al. [26] ). The wild type and the btsz K13-4 genomic regions are represented as lines with the dashed region indicating the deletion in the btsz K13-4 allele. Boxes below represent the 15 exons of btsz (black) and the organization of exons in btsz transcripts 1 (green) and 2 (blue). ( h – j ) Ability of btsz transgenes to suppress defects in btsz K13-4 mutants. The indicated transgenic constructs were expressed in the tracheal system of btsz mutant animals and various aspects of the btsz mutant phenotype were scored. The colours of the bars correspond to those in the diagram above. Genotypes of crosses and number of larvae scored: red: btl -GAL4, UAS-GFP; btsz K13-4 /TM6B, Tb ( n =17). Green: btl -GAL4, UAS-GFP; btsz K13-4 /TM6B, Tb X UAS-Btsz1; btsz K13-4 /TM6B, Tb ( n =18). Blue: btl -GAL4, UAS-GFP; btsz K13-4 /TM6B, Tb X UAS-Btsz2; btsz K13-4 /TM6B, Tb ( n =15). Error bars in h and i represent s.d.. Btsz2, but not Btsz1, suppresses the defects in branching ( h ) and the multi-lumen phenotype ( i ) of btsz K13-4 homozygous mutants ( P =5.5 × 10 −7 and 5.6 × 10 −5 respectively, by two-tailed t -test). ( j ) Ability of the same transgenes to suppress lethality of homozygous btsz K13-4 adults. If lethality of btsz K13-4 were completely suppressed, the expected proportion of homozygous mutant flies among the offspring of the cross would be 33% (the remaining 66% are heterozygous for the balancer chromosome; homozygous balancer animals die in early larval instars). Thus, about half of the mutants were rescued to viability by the transgene. Images ( a – f ) are projections of confocal image stacks. Scale bars: ( a – c left) 75 μm and ( a – c middle and right, d – f ) 20 μm. C2, region encoding the tandem C2 domains; GFP, green fluorescent protein; MBD, region encoding the Moesin binding domain; SHD, region encoding a Synaptotagmin-like-protein homology domain. Full size image Having established that Btsz is necessary specifically for the formation of the inner luminal membrane of the terminal cell, and that the failure in lumen formation is not a consequence of defective adherens junctions, we wished to determine through which intermediates it acts on the luminal membrane. One hint comes from the nature of the btsz K13-4 allele, the sequence of which predicts an mRNA lacking part of exon 8 ( Fig. 3g ), which would produce a protein without the MBD. It is not known which of the predicted btsz transcripts are present in tracheal cells. RT-PCR showed that transcripts containing exon 8 are expressed ( Supplementary Fig. S3 ). mRNA from btsz K13-4 larvae yielded a product of reduced size for exon 8 as predicted by the genomic deletion. Therefore, the form of Btsz present in btsz K13-4 mutant tracheal cells does not contain an MBD. The fact that the btsz K13-4 allele is not lethal suggests that the protein encoded by the mutant transcript is able to carry out some of Btsz’s normal functions. The observed mutant phenotype in tracheal cells might be due to either a non-specific, overall reduction of Btsz activity or, alternatively, the absence specifically of the MBD. To distinguish between these possibilities, we expressed the btsz isoforms btsz -1 (without exon 8) and btsz -2 (containing exon 8, Fig. 3g ) in the tracheal system of btsz K13-4 larvae. We found that only the MBD-containing isoform encoded by btsz -2 suppresses the mutant phenotype, even allowing homozygous mutant animals to survive and eclose as adults ( Fig. 3h–j ). This shows that the MBD is necessary for tracheal development and function. Proteins of the Ezrin-Radixin-Moesin family have been found to be associated with the morphogenesis of the inner membrane in the development of tubular organs in Drosophila [19] , [23] , [31] , C. elegans [9] , [32] , zebrafish [33] and mouse [34] . Moesin, the only member in Drosophila of the Ezrin-Radixin-Moesin family, is present at the luminal membrane in terminal cells in the embryo [23] . We found that a Moesin-GFP reporter [35] was distributed throughout the cytoplasm in terminal cell with a slight enrichment in the luminal membrane, whereas the active, phosphorylated form of Moesin (P-Moesin) was found almost exclusively at the luminal membrane ( Fig. 4a ), making it a good candidate for an effector of Btsz in luminal membrane formation. We therefore tested whether the apical localization of P-Moesin depends on Btsz and found that P-Moesin was greatly reduced or found in ectopic sites, both in btsz K13-4 mutant and in btsz -RNAi terminal cells ( Fig. 4b ; Supplementary Fig. S4 ). For comparison, the distribution of P-Moesin was not affected in Talin-depleted cells ( Supplementary Fig. S4E ), consistent with a previous report [24] . P-Moesin staining was also strongly reduced in the fusion cells in the dorsal trunk in btsz K13-4 mutant larvae ( Fig. 4d ). Thus, Btsz is required for the localization of activated Moesin in both types of tracheal cells in which we had observed defects in btsz mutants. 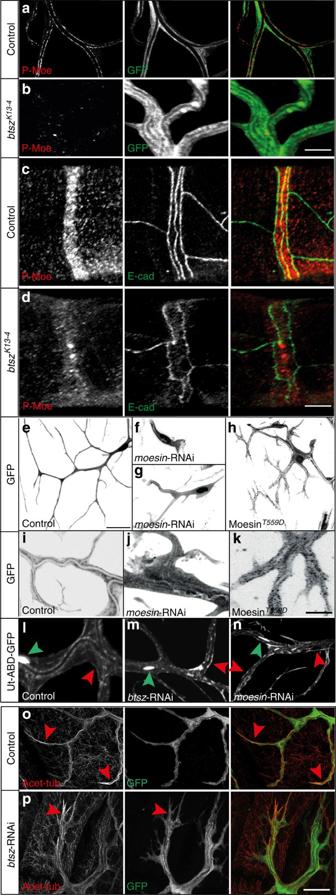Figure 4: Role of Moesin in terminal branch development. (a–d) Distribution of activated Moesin (phosphorylated form of Moesin (P-Moe)) in control andbtszK13-4mutant larvae. (a,b) Details of terminal branches expressing cytoplasmic GFP and stained with an antibody specific for the P-Moe. (a) Control larvae andbtszK13-4mutant larvae (b). (c,d) Localization of P-Moe (red) in dorsal trunk fusion cells in control (c) andbtszK13-4(d), larvae co-stained for E-cadherin (green). The images show the two ring-shaped fusion cells that connect the tracheal segments of the dorsal trunk. The apical localization of P-Moe seen in control cells is lost in thebtszK13-4mutant cells. (e–k) Effect of modulating Moesin activity in terminal cells. (e–h) Third instar terminal cells expressing cytoplasmic GFP are shown for each genotype.moesin-RNAi or MoesinT559Dwas expressed in the tracheal system using btl-GAL4. Images are colour inverted. (e) Control; (f,g)moesin-RNAi; (h) MoesinT559D. (i–k) Details of branches in control cells (i) ,moesin-RNAi (j) and MoesinT559D-expressing (k) cells at higher magnification. (l–n) Effect of loss of Moesin or Btsz on the actin cytoskeleton. Details of third instar terminal cells in which Ut-ABD-GFP was expressed as marker for actin together with RNAi specific for Btsz or Moesin. F-actin is enriched at the luminal membrane in control cells (l), and in discontinuous patches along the outer, basal membrane (red arrowhead). The marker is also seen in small irregular structures in the cytoplasm, and occasional large, smooth aggregates (green arrowhead). Afterbtszormoesindepletion, the accumulation of the marker at the luminal membrane is reduced or lost (m,n). The discontinuous patches along the outer membrane and the large aggregates are not affected (m,n). (o,p) Distribution of acetylated microtubules in terminal cells. Control (o) and Btsz-depleted (p) terminal cells in third instar larvae were stained with antibodies against acetylated tubulin. Stable acetylated microtubules extend beyond the blind end of the terminal branch lumen (red arrowhead) both in control and Btsz-RNAi cells. The RNAi constructs were co-expressed with (f,g,j,p) or without (l,m,n) Dicer2. (e–k) are of projections of confocal image stacks.l–nare single focal planes from confocal stacks. Scale bars: (e–h) 50 μm, (a,b,i–n) 10 μm and (c,d,o,p) 20 μm. GFP, green fluorescent protein. Figure 4: Role of Moesin in terminal branch development. ( a – d ) Distribution of activated Moesin (phosphorylated form of Moesin (P-Moe)) in control and btsz K13-4 mutant larvae. ( a , b ) Details of terminal branches expressing cytoplasmic GFP and stained with an antibody specific for the P-Moe. ( a ) Control larvae and btsz K13-4 mutant larvae ( b ). ( c , d ) Localization of P-Moe (red) in dorsal trunk fusion cells in control ( c ) and btsz K13-4 ( d ), larvae co-stained for E-cadherin (green). The images show the two ring-shaped fusion cells that connect the tracheal segments of the dorsal trunk. The apical localization of P-Moe seen in control cells is lost in the btsz K13-4 mutant cells. ( e – k ) Effect of modulating Moesin activity in terminal cells. ( e – h ) Third instar terminal cells expressing cytoplasmic GFP are shown for each genotype. moesin -RNAi or Moesin T559D was expressed in the tracheal system using btl-GAL4. Images are colour inverted. ( e ) Control; ( f , g ) moesin -RNAi; ( h ) Moesin T559D . ( i – k ) Details of branches in control cells ( i ) , moesin- RNAi ( j ) and Moesin T559D -expressing ( k ) cells at higher magnification. ( l – n ) Effect of loss of Moesin or Btsz on the actin cytoskeleton. Details of third instar terminal cells in which Ut-ABD-GFP was expressed as marker for actin together with RNAi specific for Btsz or Moesin. F-actin is enriched at the luminal membrane in control cells ( l ), and in discontinuous patches along the outer, basal membrane (red arrowhead). The marker is also seen in small irregular structures in the cytoplasm, and occasional large, smooth aggregates (green arrowhead). After btsz or moesin depletion, the accumulation of the marker at the luminal membrane is reduced or lost ( m , n ). The discontinuous patches along the outer membrane and the large aggregates are not affected ( m , n ). ( o , p ) Distribution of acetylated microtubules in terminal cells. Control ( o ) and Btsz-depleted ( p ) terminal cells in third instar larvae were stained with antibodies against acetylated tubulin. Stable acetylated microtubules extend beyond the blind end of the terminal branch lumen (red arrowhead) both in control and Btsz-RNAi cells. The RNAi constructs were co-expressed with ( f , g , j , p ) or without ( l , m , n ) Dicer2. ( e – k ) are of projections of confocal image stacks. l – n are single focal planes from confocal stacks. Scale bars: ( e – h ) 50 μm, ( a , b,i – n ) 10 μm and ( c,d , o , p ) 20 μm. GFP, green fluorescent protein. Full size image Depletion as well as over-activation of Moesin affected terminal cell development. Co-expression of the moesin -RNAi constructs with dicer 2 abolished branching almost completely, whereas a constitutively active, phospho-mimetic form of Moesin [35] produced short branches with disorganized lumens, in which branching points were closer together than normal ( Fig. 4f–k ). In conclusion, properly controlled Moesin activation, mediated by its interaction with Btsz at the luminal membrane, is required for proper lumen morphogenesis. Btsz and Moesin may structure the actin cytoskeleton and luminal cortical network and thereby guide membrane morphogenesis. The actin-reporter Ut-ABD-GFP is seen in patches along the outer, basal membrane, in thin strands within the cytoplasm, and in association with the luminal membrane ( Fig. 4l ). For unknown reasons, Ut-ABD-GFP also forms large aggregates, which however do not interfere with the development or function of the cells. In Btsz- or Moesin-depleted cells, the tight luminal membrane localization of the reporter-GFP was lost, whereas basally located F-actin appeared unaffected ( Fig. 4m,n ). Btsz and Moesin are therefore specifically required for the organization of the lumen-associated actin cytoskeleton in terminal cells. One function of an apical, cortical actin cytoskeleton is the cortical organization of microtubules. The growth of the tracheal tube in fact depends on the microtubule cytoskeleton [20] , [21] , and it was therefore possible that an indirect effect of Btsz and Moesin on microtubules was partly responsible for the defects. We found that the track of acetylated, stable microtubules that is formed ahead of the growing tip of the lumen [1] , [21] was intact both in the embryo and in the larva ( Fig. 4p ). Thus, the tracks that are thought to guide the growth of the lumen were present. We conclude that the defects seen in the absence of Btsz or Moesin are not caused by an indirect effect of the actin cytoskeleton on microtubule function. The cortical actin cytoskeleton also has a role in secretion, which in tracheal cells is necessary for the expansion and maturation of the multicellular tracheal lumen [36] . However, we found no indication that the coupling of the secretory pathway to the luminal membrane was impaired in Btsz- or Moesin-depleted cells. Even the abnormal lumens in such cells contain secreted chitinous material (tested in the embryo, Fig. 6f,g ), were filled with gas and reflected light (seen in the larva; Supplementary Fig. S2 ). These are indications that the materials needed for lumen maturation were being properly secreted. 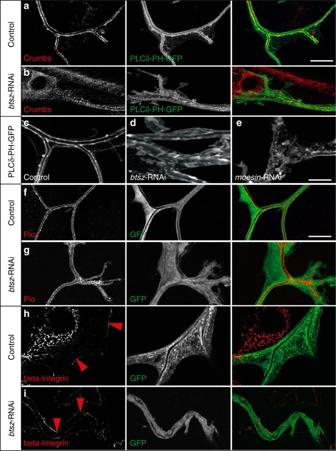Figure 5: Apical membrane markers and secretion in Btsz-depleted terminal cells. (a,b) Terminal cells expressing PLCδ-PH-GFP (green) were stained with antibodies against Crumbs (red). Crumbs is apically enriched in control (a) but not inbtsz-RNAi (b). Localization of PLCδ-PH-GFP in control (a,c),btsz-RNAi (b,d) andmoesin-RNAi (e) terminal cells. Apical localization of PLCδ-PH-GFP is disrupted inbtsz-RNAi (b,d) andmoesin-RNAi (e) cells. Distribution of Pio (red) in control (f) andBtsz-depleted (g) cells. Localization of β-integrin (red arrowhead inh,i) to the outer membrane in control cell (h) and in Btsz-depleted cells (i). (c–e) and (h,i) are single focal planes from confocal stacks and (a,b) and (f,g) are projections of confocal image stacks. Scale bars: (a,b,f–i) 10 μm, (c–e) 5 μm. Figure 5: Apical membrane markers and secretion in Btsz-depleted terminal cells. ( a , b ) Terminal cells expressing PLCδ-PH-GFP (green) were stained with antibodies against Crumbs (red). Crumbs is apically enriched in control ( a ) but not in btsz- RNAi ( b ). Localization of PLCδ-PH-GFP in control ( a , c ), btsz- RNAi ( b , d ) and moesin- RNAi ( e ) terminal cells. Apical localization of PLCδ-PH-GFP is disrupted in btsz -RNAi ( b , d ) and moesin -RNAi ( e ) cells. Distribution of Pio (red) in control ( f ) and Btsz -depleted ( g ) cells. Localization of β-integrin (red arrowhead in h , i ) to the outer membrane in control cell ( h ) and in Btsz-depleted cells ( i ). ( c – e ) and ( h , i ) are single focal planes from confocal stacks and ( a , b ) and ( f , g ) are projections of confocal image stacks. Scale bars: ( a , b , f – i ) 10 μm, ( c – e ) 5 μm. 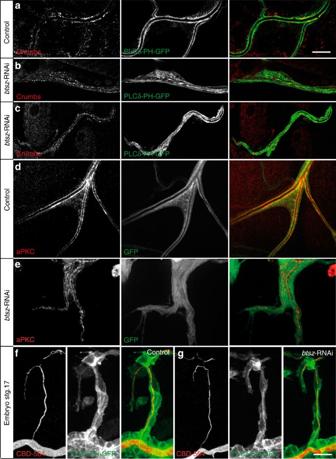Figure 6: Localization of apical and secreted proteins in terminal cells. (a–c) Crumbs localization in control (a) and Btsz-depleted (b,c) larval terminal cells; single focal planes. (d,e) Larval terminal cells expressing cytoplasmic GFP (green) were stained with antibodies against aPKC (red). aPKC remains associated with the luminal membrane after Btsz depletion (e). (f,g) Luminal chitin deposition in control (f) andbtsz-RNAi (g) dorsal terminal cells in the embryo. Embryos expressing PLCδ-PH-GFP (green) were stained with the chitin-interacting dye CBD-564. Scale bars: (a–e) 10 μm, (f,g) 5 μm. Full size image Figure 6: Localization of apical and secreted proteins in terminal cells. ( a – c ) Crumbs localization in control ( a ) and Btsz-depleted ( b , c ) larval terminal cells; single focal planes. ( d , e ) Larval terminal cells expressing cytoplasmic GFP (green) were stained with antibodies against aPKC (red). aPKC remains associated with the luminal membrane after Btsz depletion ( e ). ( f , g ) Luminal chitin deposition in control ( f ) and btsz -RNAi ( g ) dorsal terminal cells in the embryo. Embryos expressing PLCδ-PH-GFP (green) were stained with the chitin-interacting dye CBD-564. Scale bars: ( a – e ) 10 μm, ( f , g ) 5 μm. Full size image Delivery of apical cargo to the luminal membrane Since the luminal membrane-associated F-actin is disrupted, and the lumen is not properly formed in Btsz-depleted cells, Btsz, Moesin and actin must be required in some manner for the assembly of the tube. We looked into this using three markers for the luminal membrane, the apical transmembrane protein Crumbs, which is present in tubes from their earliest appearance on, the transmembrane protein Pio [37] , a later marker for mature luminal membrane [37] , and PLCδ-PH-GFP. In control cells, Crumbs is associated with the luminal membrane in a punctate manner ( Fig. 5a ; Fig. 6a ). In Btsz-depleted cells, we see a lower level and less regular distribution of Crumbs in the luminal membrane ( Fig. 5b ; Fig. 6b,c ), suggesting that Crumbs-containing membrane is not delivered efficiently. By contrast, the delivery of a basal transmembrane protein, the β-chain of the integrins, to the outer membrane was not affected after depletion of Btsz ( Fig. 5i ). Both Btsz- and Moesin-depleted cells also showed abnormalities in the distribution of PLCδ-PH-GFP, with positive patches of various sizes that were not associated with the lumen ( Fig. 5b,d,e ). We wondered whether the larger PLCδ-PH-GFP-positive structures might be parts of the luminal membrane that had either not been assembled properly or had disintegrated. In Btsz-depleted cells, Pio was seen only in association with the lumen and not in vesicles or elsewhere in the cell ( Fig. 5f,g ). Similarly, the localization of an apical membrane-associated protein, aPKC, showed no significant irregularity in Btsz-depleted cells ( Fig. 6e ). Thus, the secretory path associated with membrane maturation is not affected, nor do the PLCδ-PH-GFP structures in the cytoplasm represent fragments of mature tubes. Instead, it seems more likely that the PLCδ-PH-GFP-positive patches represent membrane that has not been incorporated into the apical membrane forming the lumen. The actin cytoskeleton performs many functions in tracheal cells that are regulated by different actin-binding proteins. F-actin is present in the growth-cone-like leading tip during branch extension [1] , [23] ( Fig. 2c ), it stabilizes the anchorage of mature branches on the extracellular matrix via integrins [24] , and a network of filamentous actin also surrounds the lumen. While mediators for the filopodial and the basal actin functions have been identified previously (Ena and Talin), and one function of the apical cytoskeleton depends on Diaphanous, we show here that Btsz selectively organizes or stabilizes the apical actin domain and the apical membrane in the tracheal terminal cell. In the embryonic epithelium [27] and in multicellular epithelial tubes [29] , the major role of Btsz is to stabilize adherens junctions. The physical distance between adherens junctions and the growing apical domain in distant branches of terminal cells, and the intact adherens junctions in many severely malformed mutant cells indicate that the role of Btsz in terminal cells is separable from a potential influence on adherens junction stability. The selective defects in apical membrane organization caused by Btsz depletion might be due to failures in any of the various functions of the apical actin cortex, including structural support for the developing tube membrane, trafficking membrane and protein material destined for the tube or facilitating fusion of the vesicles with the tube membrane. Two members of the mammalian SLP family have been found to be needed for de novo lumen formation in a multicellular tube [28] . While Btsz has been referred to as an SLP family member, many of the predicted transcripts in fact lack the exon encoding a motif that is characteristic for vertebrate SLPs, the SLP family homology domain. We show that transcripts encoding this domain are present in tracheal cells ( Supplementary Fig. S3 ), and the function we describe here for Btsz may be related to the vesicle-trafficking roles of SLP family members in vertebrates. We cannot exclude a role for Btsz/Moesin and actin in the structural support of the tube, but the presence of PLCδ-PH-GFP-containing vesicles in the cytoplasm of Btsz-depleted cells indicates that Btsz deficiency affects the trafficking or assembly of membrane material. It is certainly the case that there is more than one path from the Golgi to the tube membrane. Both Crumbs and Pio are transmembrane proteins, thus both must be delivered through the Golgi, and indeed apical secretion into the tracheal lumen has been shown to occur through distinct pathways characterized by specific cargoes and mediator s [36] . One path delivers chitin-modifying enzymes and targets them to septate junctions. Another path requires the apical actin cytoskeleton and delivers 2A12 and Pio in a Diaphanous- and Rho1-dependent manner. A third path has been postulated to be responsible for the delivery of apical membrane proteins such as Crumbs that is independent of Diaphanous and septate junctions. Our results here show that in terminal cells Btsz and Moesin are involved in this pathway. Pio localization is normal in mature tubes that have managed to develop in Btsz-depleted cells, whereas Crumbs is reduced. This suggests that Btsz is required for a pathway delivering a specific subset cargo to build the apical domain, one that depends on the F-actin cortex around the tube, and includes the apical determinant Crumbs. Fly stocks Throughout this work we used the btl -GAL4 driver line to express UAS transgenes and RNAi constructs in the tracheal system. w[1118]; P{ ry [+t7.2] neoFRT}82B, btsz K13-4 /TM3, Sb 1 , w[1118]; P{ ry [+t7.2] neoFRT}82B btsz J5-2 /TM3, Sb 1 , w[1118]; P{w[+mC]=GUS-Btsz.2polyG}2, w[1118]; P{w[+mC]=GUS-Btsz.1}2, w[1118]; P{w[+mC]=UAS-Moe.T559D.MYC}2, w[1118]; P{w[+mC]=UAS-Moe.IR.327-775}3, w[*]; P{w[+mC]=UAS-Rho1.V14.E40L}4 and w[*]; P{w[+mC]=UAS-Rho1.N19}2.1 were obtained from the Bloomington stock centre. UAS-Btsz2-ΔC2-HA, UAS-Ut-ABD-GFP, UAS-PLCδ-PH-GFP and btsz K13-4 /TM3, Sb 1 KrG4-UAS-GFP from Thomas Lecuit. RNAi transgenes from the VDRC stock center: btsz (102608, 35205, 35206), moesin (37917, 110654), talin (40399,40400), rho1 (109420, 12734) and UAS- dicer 2 (60008). RNAi transgenes from the NIG stock centre: btsz (7343R-1) and moesin (10701R-1). For the rescue experiments, GUS-Btsz1 and GUS-Btsz.2polyG. were crossed into btsz K13-4 /TM6B, Tb background and homozygous btsz K13-4 mutant larvae were identified by selecting Tb + larvae. Antibodies used in immunostainings The following primary antibodies were used: rabbit anti-Glu-Glu tag (anti-polyomavirus epitope mouse antibodies, 1:200, Cell Signaling), rat anti-HA (1:100, Boehringer Mannheim), rabbit anti-Dof (1:200 (ref. 38 )), rabbit anti-P Moe (1:250, Cell Signaling), rat anti-Crumbs (1:100, gift from Elisabeth Knust), rabbit anti-Pio (1:300 (ref. 34 )), mouse anti β-Integrin (1:200, DSHB), rabbit anti-aPKC (1:200, Santa Cruz), mouse anti-Rho1 (1:100, DSHB) and rabbit anti-GFP (1:500, Torrey Pines Biolabs Inc.). Fluorochrome (Alexa468, Alexa568 and Alexa647)-conjugated secondary antibodies (Molecular Probes) were used at a dilution of 1:500. Chitin binding probe-fluorochrome conjugate production The SNAP-CBD (NEB, plasmid pYZ205) was expressed in T7 express cells (NEB, C2566), purified and conjugated with SNAP-Surface Alexa Fluor564 and SNAP-Surface Alexa Fluor647. The SNAP-CBD purification and conjugation with fluorochromes were performed according to the SNAP-Fusion protocol provided by NEB. The CBP-fluorochrome conjugates were tested in embryos using a standard staining protocol [38] and used at a final concentration of 1:300. Sample preparation and microscopy Third instar larvae were filleted and fixed with 4% paraformaldehyde for 20 min. Fixed fillets were washed with 0.3% PTX (PBS+0.3% Triton X-100) three times for 10 min each followed by 1 h incubation in blocking reagent (0.3% PTX+1% bovine serum albumin). After blocking, the fillets were incubated overnight in antibody solution at 4 °C, washed 4 times (15 min each) in 0.1% PTX, incubated in Alexa-conjugated secondary antibodies for 2 h at room temperature, then washed for 2 h at room temperature and mounted in Vectashield. Leica TCS SP2, Zeiss Apotome and Leica M2 16FA were used for microscopy. Images were acquired using the software packages Leica Confocal Software LCS, Axiovision Rel 4.6 (Zeiss) and Axiovision 1 (Zeiss), and edited using Adobe Photoshop (Adobe Systems) and ImageJ software. Microsoft Office Excel was used for graphs and statistical analysis. Time–course studies For the time–course analysis, larvae of appropriate genotype and stages (first instar, 24 h; second instar, 44 h; mid-third instar, 96 h; late third instar, 110 h after egg lay) were collected, rinsed in PBS and anesthetised using a 1:1 solution of chloroform and halocarbon oil. The anaesthetised larvae were mounted in chloroform/halocarbon oil and imaged using a Leica TCS SP2 confocal microscope. Terminal branches of the dorsal terminal cells (between tracheal segments tr2 to tr9) were counted, and statistical analysis were performed using Microsoft Excel and Prism6 softwares. Time-lapse imaging Embryos for live imaging were dechorionated in 4% bleach and mounted on a glass coverslip in halocarbon oil. Time-lapse experiments were carried out either on a PerkinElmer UltraVIEW VoX or an UltraVIEW ERS spinning disc confocal microscope. Dorsal terminal cells from tr5 to tr9 segments were analysed by collecting Z stacks at 0.6 or 1 μm thickness at 2-min time intervals. Measurement and quantification of the ratio between lumen and cell length Staged (stage 16–17) embryos were collected, fixed and stained using standard protocols [38] . Anti-GFP antibody and CBP-Alexa564 were used for visualizing the terminal cells and tubes, respectively. The samples were imaged using a Leica TCS SP2 confocal microscope. The tube length was measured between the point of origin of the terminal cell tube (from the dorsal branch tube) and its distal tip. The cell length was calculated by extending the second point (from the tip of the tube) to the tip of the leading edge of the outer membrane. The images were processed using ImageJ, the measurements were taken using the NeuronJ plugin and the statistical analyses were performed using Microsoft Excel and Prism6 softwares. RT-PCR experiments For the RT-PCR experiments, RNA was extracted using Trizol (Invitrogen Life Technologies) either from whole larvae or tracheal cells isolated manually from third instar larvae. The exons were amplified from complementary DNA using the primers shown in Supplementary Table S1 . How to cite this article: JayaNandanan, N. et al. Guidance of subcellular tubulogenesis by actin under the control of a synaptotagmin-like protein and Moesin. Nat. Commun. 5:3036 doi: 10.1038/ncomms4036 (2014).